Integrated photosystem II-based photo-bioelectrochemical cells Photosynthesis is a sustainable process that converts light energy into chemical energy. Substantial research efforts are directed towards the application of the photosynthetic reaction centres, photosystems I and II, as active components for the light-induced generation of electrical power or fuel products. Nonetheless, no integrated photo-bioelectrochemical device that produces electrical power, upon irradiation of an aqueous solution that includes two inter-connected electrodes is known. Here we report the assembly of photobiofuel cells that generate electricity upon irradiation of biomaterial-functionalized electrodes in aqueous solutions. The cells are composed of electrically contacted photosystem II-functionalized photoanodes and an electrically wired bilirubin oxidase/carbon nanotubes-modified cathode. Illumination of the photoanodes yields the oxidation of water to O 2 and the transfer of electrons through the external circuit to the cathode, where O 2 is re-reduced to water. Photosynthesis is a sustainable effective and a complex process that converts light energy into chemical energy that is stored in fuel products [1] , [2] , [3] , [4] . The photosynthetic apparatus operates through the coupled excitation of two reaction centres (RCs) consisting of photosystems I and II, PSI and PSII. Photoexcitation of PSI leads to an electron transfer to the ferredoxin units, which leads ultimately to the production of NADPH that activates the Calvin cycle and the fixation of CO 2 to sugars [5] . The photoexcitation of PSII results in the electron transfer to the quinone, Q A , acceptor that stimulates the reduction of plastoquinone-9, which, through a series of electron-transfer processes, regenerates PSI. The oxidized species generated in PSII oxidizes the Mn 4 O 5 complex that catalyses the oxygen evolution while regenerating the PSII centre [6] , [7] . Recently, extensive research efforts were directed towards the development of photoelectrochemical or solar cells mimicking photosynthesis [8] , [9] , [10] , [11] , [12] , [13] , or to the application of the native photosystems to power photoelectrochemical cells. For example, dye-sensitized solar cells that include synthetic photosensitizers and enzymes were reported, and the resulting hybrid systems were implemented to generate the hydrogen fuel [14] , or photocurrents [15] . Nonetheless, in these systems the cathodic reactions were not directly coupled to the product generated at the photoanodes, resulting in a waste product. Also, different microbial photobiofuel cells (PBFCs), which use whole-cell bacteria that upon photoirradiation generate fuel products providing the source for electrical power, were reported [16] , [17] , [18] . Different bioelectrochemical devices that implement the RC, PSI and/or PSII as light harnessing components for the activation of PBFCs producing photocurrents [19] , [20] , [21] , [22] , or fuel products [23] , [24] , [25] have been proposed. These PBFCs require the immobilization and electrical contacting of the light harnessing components with the electrode supports to the extent that photo-induced electron-transfer processes occur between the photosynthetic RC, thus enabling the generation of photocurrents (or their use for the synthesis of fuel products). The electrical contacting of redox proteins with electrodes attracted substantial research efforts directed to the development of amperometric biosensors [26] , [27] , [28] , [29] or biofuel cell elements [30] , [31] , [32] , [33] , [34] , [35] . Different methods to integrate redox proteins with electrodes in electrically contacted configurations were developed, including the modification of the proteins with relay units [36] , [37] , the reconstitution of the proteins on relay-cofactor units [38] , [39] , [40] and the immobilization of the proteins in redox-active polymer matrices [41] . Related principles were implemented to electrically wire PSII with electrode surfaces. For example, PSII was deposited on a mercapto benzoquinone monolayer assembled on a Au electrode for sensing applications [42] . Photoexcitation of the complex that mimicked the native PSII/Q A complex resulted in O 2 evolution with the generation of photocurrent. Similarly, the PSII was electrically contacted with electrode surfaces by its immobilization in polymer hydrogels consisting of the Os(II/III)-polypyridine complex as electron transfer relay units [43] . Electrical wiring of PSI with electrodes was demonstrated by the reconstitution of the native PSI, from which vitamin K 1 was excluded, onto a synthetic quinone acceptor linked to a functionalized electrode by electrostatic interactions [44] . Similarly, iron-sulfur cluster-modified Au or Pt nanoparticles (NPs) were reconstituted into apo-PSI, resulting in the wiring, and H 2 evolution by the hybrid system [45] . Furthermore, the genetically engineered photosynthetic RC was oriented in a monolayer configuration on electrode supports using a His-tag Ni-NTA complex, and the resulting photocurrents in the presence of an electron mediator, were monitored [46] , [47] . Also, alignment of PSI on electrode surfaces was achieved with the aid of bis-aniline-crosslinked Pt nanoclusters [48] or by using redox polymer matrices as electron-transfer relays [21] . Although the generation of photocurrents was demonstrated in these systems, in all cases a potentiostat was used as a sink (or source) for the electrons, and sacrificial electron donors or acceptors had to be included in the system to generate steady-state currents. To date, no integrated photo-bioelectrochemical device (bio-photovoltaic cell) that produces electrical power upon illumination of two inter-connected electrodes is known. Here we report the assembly of an integrated PBFC composed of a PSII-modified electrode, acting as a photoanode for the light-induced oxidation of H 2 O to O 2 , and a bilirubin oxidase/carbon nanotubes (BOD/CNTs)-functionalized electrode acting as a cathode for the reduction of O 2 to H 2 O. Illumination of this cell results in the formation of electricity, in the absence of any added sacrificial reagent. A PSII/benzoquinone polymer-based photo-bioelectrochemical cell We have implemented PSII isolated from the theromphilic cyanobacterium Mastigocladus laminosus ( Supplementary Figs S1–S4 ). The PBFC is schematically presented in Fig. 1 . The photoanode was prepared by the primary electropolymerization of mercapto benzoquinone on a Au surface, effective illuminated area ca 0.13 cm 2 . The resulting poly(mercapto- p -benzoquinone), pMBQ, matrix showed a quasi-reversible redox-wave at E °′=−0.05 V versus a KCl-saturated calomel electrode (SCE), pH=7.4. The current peak value of the redox-wave revealed a linear dependence with the scan rate, consistent with a surface-confined redox system. The surface coverage of the quinone units on the electrode corresponded to 4.7×10 −9 mol cm −2 (for the electrochemical characterization of the pMBQ matrix, see Supplementary Fig. S5 ). PSII was, then, deposited onto the quinone layer with the vision that the quinone units would bind to the Q B site of PSII and act as electron mediators that electrically wire the PSII with the electrode. The PSII associated with the polymer was, subsequently, crosslinked by bis[sulfosuccinimidyl] suberate (BS 3 ) to yield the integrated photoanode. Microgravimetric quartz-crystal microbalance measurements indicated a surface coverage of PSII that corresponded to 1.5×10 −12 mol cm −2 . Knowing the dimensions of the PSII [7] , this value translates to ca 53% of a random densely packed monolayer. Figure 2a shows the photocurrent action spectra upon illumination of the electrode in a pure buffer solution. 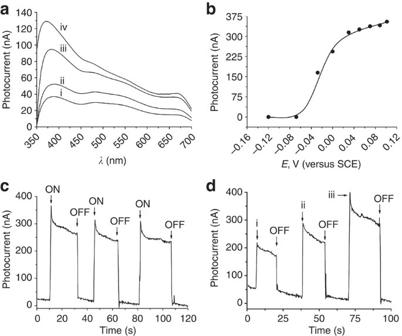Figure 2: Operation of the poly(mercapto-p-benzoquinone)/photosystem II anode. (a) Photocurrent action spectra corresponding to the pMBQ/PSII anode following the electropolymerization atE=0.6 V versus saturated calomel electrode (SCE) for: (i) 500, (ii) 1,000, (iii) 2,000 and (iv) 3,000 s. (b) Dependence of the photocurrent on the external potential applied on the pMBQ/PSII anode.P=0.10 W,λ>400 nm. (c) Photocurrent responses of the pMBQ/PSII anode to repetitive illumination and darkness cycles. Potential appliedE=0.15 V versus SCE,P=0.10 W (lamp power intensity atλ>400 nm). (d) Photocurrent responses of the pMBQ/PSII anode to repetitive illumination (at variable intensities) and darkness cycles. The illumination,λ>400 nm, intensities are: (i)P=0.04, (ii)P=0.07 and (iii)P=0.10 W. Potential applied:E=0.15 V versus SCE. All measurements were performed in a phosphate buffer solution (0.1 M, pH=7.4). The photo-induced quinone-mediated electron transfer to the electrode, and the concomitant oxidation of water to O 2 , yield the observed photocurrent. The photocurrent action spectrum follows, as expected, the spectral features of PSII. Also, the intensities of the photocurrent are controlled by the duration of the electrodeposition process applied to polymerize the polymer. The photocurrents are intensified upon applying the electropolymerization potential (0.6 V versus SCE) for a time-interval of 50 min, and then level off to a saturation value. Further application of the potential for 15 min caused a 20% decrease in the photocurrent. The effect of the time-interval of electropolymerization on the resulting photocurrents might be attributed to the charge transport functions of the polymer matrix in improving the electrical contacting efficiency of PSII with the electrode. In the first phase of electropolymerization (up to 50 min), an optimal coverage of the electrode with the charge transporting polymer film takes place. 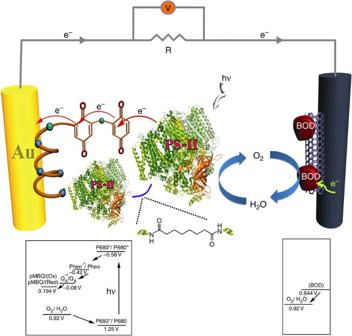Increasing the thickness of the polymer by further electropolymerization perturbs the charge transport properties of the film due to the existence of defects in the polymer matrix, which results in lower photocurrent values. Figure 1: Schematic presentation of the poly(mercapto-p-benzoquinone)/photosystem II/bilirubin oxidase/carbon nanotubes photoelectrochemical cell. The protein structure was originally published in ref.60. Copyright, The American Society for Biochemistry and Molecular Biology. The insets depict the energy diagrams associated with the components of the cell. Figure 1: Schematic presentation of the poly(mercapto- p -benzoquinone)/photosystem II/bilirubin oxidase/carbon nanotubes photoelectrochemical cell. The protein structure was originally published in ref. 60 . Copyright, The American Society for Biochemistry and Molecular Biology. The insets depict the energy diagrams associated with the components of the cell. Full size image Figure 2: Operation of the poly(mercapto- p -benzoquinone)/photosystem II anode. ( a ) Photocurrent action spectra corresponding to the pMBQ/PSII anode following the electropolymerization at E =0.6 V versus saturated calomel electrode (SCE) for: (i) 500, (ii) 1,000, (iii) 2,000 and (iv) 3,000 s. ( b ) Dependence of the photocurrent on the external potential applied on the pMBQ/PSII anode. P =0.10 W, λ >400 nm. ( c ) Photocurrent responses of the pMBQ/PSII anode to repetitive illumination and darkness cycles. Potential applied E =0.15 V versus SCE, P =0.10 W (lamp power intensity at λ >400 nm). ( d ) Photocurrent responses of the pMBQ/PSII anode to repetitive illumination (at variable intensities) and darkness cycles. The illumination, λ >400 nm, intensities are: (i) P =0.04, (ii) P =0.07 and (iii) P =0.10 W. Potential applied: E =0.15 V versus SCE. All measurements were performed in a phosphate buffer solution (0.1 M, pH=7.4). Full size image The effect of applied potential on the resulting photocurrent is displayed in Fig. 2b . Although at potentials higher than E =0.0 V versus SCE the photocurrents reveal a high value, >300 nA, lowering the applied potential below E =0.0 V sharply decreases the photocurrents. This is consistent with the redox potential of the pMBQ matrix, E°′~−0.05 V versus SCE. At positive potentials, the relay units are retained in their oxidized quinoid state, and thus, the photo-induced electron transfer is accompanied by an immediate pumping of the electrons from the relay units to the electrode (the PSII is wired with the electrode by means of the pMBQ polymer). This vectorial electron transfer minimizes back electron transfer reactions and leads to high photocurrents. As the potential turns negative, the relay units are transformed into the hydroquinone state that does not accept the electrons from the PSII. As a result, the transfer of electrons from the protein to the electrode is perturbed, leading to the recombination of the electron-hole species, and to substantially lower photocurrents. Figure 2c shows the switchable generation of the photocurrent upon a cyclic 'ON-OFF' illumination of the photoanode. Evidently, the intensity of the photocurrent is controlled by the light intensity implemented to illuminate the photoanode ( Fig. 2d ). The cathode of the photo-bioelectrochemical cell consisted of a composite of BOD and oxidized CNTs deposited onto a glassy carbon (GC) electrode. The deposition of BOD on the CNTs was found to electrically contact the enzyme with the bulk electrode, resulting in the bioelectrocatalysed reduction of O 2 to water (see Supplementary Fig. S6 ). These bioelectrocatalytic functions of the BOD/CNTs were previously implemented to develop biofuel cells using glucose [49] , [50] or ethanol [49] as fuels. Accordingly, the pMBQ/PSII photoanode was coupled to the BOD/CNTs cathode ( Fig. 1 ). Irradiation of the photoanode under air resulted in the formation of a photocurrent. The current–voltage discharge curve of the photo-electrochemical cell at variable resistances is displayed in Fig. 3a , and the power output is shown in Fig. 3b . Control experiments revealed that minute currents were generated in the dark. Also, irradiation of the system under an inert Ar atmosphere resulted in a small current, which may be attributed to the formation of O 2 at the photoanode, or its possible leakage into the system. In a further experiment, the thermal denaturation of BOD blocked the formation of the photocurrent upon irradiation of the system under O 2 . These control experiments imply that the pMBQ/PSII photoanode and the BOD/CNTs cathode indeed yield an integrated system, where the photo-oxidation of water to O 2 proceeds at the anode concurrently with the reduction of O 2 at the cathode. Furthermore, the current generated by the system remained fairly constant for a time-interval of 3 h of continuous irradiation and then degraded by 15% upon irradiation for 10 h. Knowing the surface coverage of PSII and the current density at the maximum power of the cell, we estimate the electron transfer turnover rate between PSII and the electrode to be 518 e − s −1 . This value is very similar to the turnover rate observed for PSII in a monolayer configuration [51] , suggesting that immobilization of PSII on the polymer matrix does not affect its activity. The PSII isolated from the theromphilic bacteria revealed an encouraging stability reflected by an activity degradation of ca 20% upon its storage at 4 °C for 2 weeks. This suggests that the future immobilization of PSII in protecting polymer matrices or its further genetic manipulation might lead to stable cell configurations. The quantum yield for the generation of the photocurrent at λ =675 nm corresponded to 1.0%. Previous studies reported on photosynthetic photoelectrochemical cells that revealed photoconversion efficiencies in the range of 0.2–3.3% (refs 52 , 53 ). Nonetheless, these systems have implemented whole photosynthetic cells and diffusional electron-transfer mediators. The advantages of our system rest on the facts that the components are fully integrated with the electrode supports, and no diffusional electron-transfer mediator must be solubilized in the electrolyte solution. Also, dye-sensitized solar cells provide an alternative, related, configuration for the conversion of light energy to electrical power [54] . This method was substantially advanced in the last two decades, and efficiencies of up to 12% were reported [55] . These systems include, however, a diffusional mediator that does not exist in our cell. Furthermore, one may use the high-surface-area deposition paradigm existing in the dye-sensitized solar cells to immobilize the PSII and BOD biocomponents for enhancing the photoconversion efficiencies. 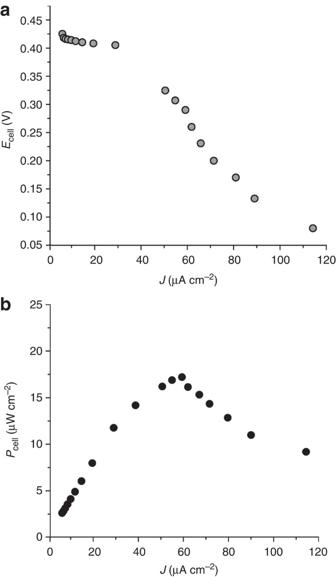Figure 3: Discharge of the poly(mercapto-p-benzoquinone)/photosystem II/bilirubin oxidase/carbon nanotubes photobiofuel cell. Cell discharge (polarization) curve (a), and the dependence of the cell power (b) on the discharge current density of the pMBQ/PSII/BOD/CNTs photobiofuel cell.P=0.10 W,λ>400 nm. Measurements were performed in air and using variable external resistances. The electrolyte was a phosphate buffer (0.1 M, pH=7.4). Figure 3: Discharge of the poly(mercapto- p -benzoquinone)/photosystem II/bilirubin oxidase/carbon nanotubes photobiofuel cell. Cell discharge (polarization) curve ( a ), and the dependence of the cell power ( b ) on the discharge current density of the pMBQ/PSII/BOD/CNTs photobiofuel cell. P =0.10 W, λ >400 nm. Measurements were performed in air and using variable external resistances. The electrolyte was a phosphate buffer (0.1 M, pH=7.4). Full size image A PSII/bis-aniline-crosslinked Au NPs photo-bioelectrochemical cell Our approach was extended to construct an integrated photoanode consisting of bis-aniline-crosslinked Au NPs and PSII, Fig. 4a . Au NPs, 3.5 nm diameter, modified with mercaptoethane sulphonic acid and mercaptoaniline were electropolymerized onto a mercaptoaniline monolayer-modified Au surface [56] , [57] , [58] . The PSII was deposited onto the Au NPs composite, and subsequently, the PSII was crosslinked with BS 3 to yield the integrated electrode (surface coverage ca 8.5×10 −13 mol cm −2 ). The bis-aniline bridging units exhibit quasi-reversible redox features, E°~0.1 V versus SCE at pH=7.4, and are oxidized at E >0.1 V to the quinoid electron acceptor state. 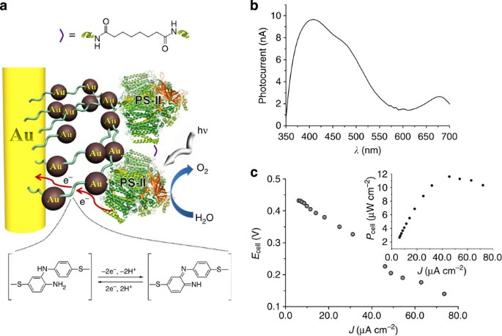Figure 4: Operation of the bis-aniline-crosslinked Au nanoparticles/photosystem II-based photoanode and biofuel cell. (a) Schematic presentation of the bis-aniline-crosslinked Au NPs/PSII anode. (b) Photocurrent action spectrum corresponding to the bis-aniline-crosslinked Au NPs/PSII anode. (c) Cell discharge (polarization) curve for the bis-aniline-crosslinked Au NPs/PSII/bilirubin oxidase/carbon nanotubes (BOD/CNTs) photobiofuel cell. Inset: the dependence of the cell power on the discharge current density.P=0.1 W,λ>400 nm. Measurements were performed in air and using variable external resistances. The electrolyte was a phosphate buffer (0.1 M, pH=7.4). Figure 4b shows the photocurrent action spectrum generated by the electrode, and Supplementary Fig. S7 depicts the effect of the applied potential on the resulting photocurrent. Evidently, at potentials E >0.1 V, where the bridging units exist in the quinoid state, high photocurrent values are observed, whereas at potentials lower than E =0.1 V, a sharp decrease in the photocurrent is detected. These results are consistent with the fact that the quinoid acceptor state of the bridging units acts as a wiring relay for transferring the electrons from the PSII to the electrode. The integrated photoanode was coupled to the BOD/CNTs cathode to yield the respective PBFC. Figure 4c depicts the photocurrent action spectrum of the cell. The power output at different external resistances is shown in Fig. 4c , inset. The quantum yield, at λ =675 nm, corresponded to ca 0.7%. It should be noted that despite the porous morphology associated with the bis-aniline-crosslinked Au NPs composite, the loading of PSII on this matrix is ca 45% lower in comparison with the pMBQ/PSII film. This may be attributed to the enhanced binding affinity of the benzoquinone units to the Q B site of the PSII, thus allowing the concentration of the photoactive component on the surface. Figure 4: Operation of the bis-aniline-crosslinked Au nanoparticles/photosystem II-based photoanode and biofuel cell. ( a ) Schematic presentation of the bis-aniline-crosslinked Au NPs/PSII anode. ( b ) Photocurrent action spectrum corresponding to the bis-aniline-crosslinked Au NPs/PSII anode. ( c ) Cell discharge (polarization) curve for the bis-aniline-crosslinked Au NPs/PSII/bilirubin oxidase/carbon nanotubes (BOD/CNTs) photobiofuel cell. Inset: the dependence of the cell power on the discharge current density. P =0.1 W, λ >400 nm. Measurements were performed in air and using variable external resistances. The electrolyte was a phosphate buffer (0.1 M, pH=7.4). Full size image The present study has introduced a new approach to construct integrated photo-bioelectrochemical cells. The novelty of the system rests on the fact that the irradiation of the biomaterial-functionalized electrodes in the aqueous solution leads to the generation of electrical power without the addition of any sacrificial reagent. The systems consist of an electrically wired PSII photoanode that photoinduces electron injection into the electrode while oxidizing water to O 2 . The electrons injected into the electrode are used for the biocatalysed reduction of O 2 at the cathode (which is composed of electrically wired BOD). The resulting photocurrents and electrical power, however, are quite low, due to three main possible reasons: (i) The surface coverage of PSII on the photoanode is low, and corresponds to 1.5×10 −12 mol cm −2 (for the pMBQ/PSII system) and 8.5×10 −13 mol cm −2 (for the bis-aniline-crosslinked Au NPs/PSII system). These values translate to ca 53 and 30% coverage of a random densely packed monolayer of PSII in the two systems, respectively. (ii) The PSII units are not optimally oriented on the quinone (or bis-aniline-bridged Au NPs) matrices, and thus, the electrical contacting of PSII with the electrodes is not optimized. As a result, charge transported to the electrodes competes inefficiently with the recombination reactions in PSII. (iii) The potential difference between the anode and the cathode of the cell is relatively low, and a substantial loss in the potential accompanies the electron transfer from PSII to the redox polymer. These limitations can be solved by increasing the content of PSII on the photoanode, and by enhancing the electrical wiring efficiency between PSII and the electrode [13] . The content of PSII on the electrode might be increased by the construction of multilayers of electrically contacted PSII, or by the roughening of the electrode surface. The enhancement of the electrical wiring efficiency between PSII and the electrode might be accomplished by nano-engineering and alignment of PSII onto the charge mediator units, for example, by the reconstitution [40] of the protein on the quinone units. The potential difference between the anode and the cathode, and thus, the power output of the photo-bioelectrochemical cell, could be improved by the chemical tuning of the redox potential associated with the electron-mediating redox polymer, to a value that is close to the potential of the Q B site. Chemicals BOD (E. C. 1.3.3.5, from Myrothecium Verrucaria , activity of 5 U mg −1 solid), was purchased from Sigma. The enzyme was used without any further purification. Single-walled CNTs, SWCNTs, with an average diameter of ca 2 nm were purchased from Nanoport (Shenzhen, China). The SWCNTs were refluxed in 2.5 M HNO 3 for 10 h, and were then washed in water and precipitated using a centrifuge to yield an average length of 2 μm. Ultrapure water from a Nanopure (Barnstead) source was used throughout this work. Mercapto benzoquinone, MBQ, was synthesized according to a previously reported method [59] . Au NPs functionalized with 2-mercaptoethane sulphonic acid and p -aminothiophenol were prepared according to a previously reported procedure [56] . The average size of the NPs was estimated by transmission electron microscope to be 3.5 nm. Extraction and purification of PSII About 60 g of the thermophilic cyanobacterium Mastigocladus laminosus cells were suspended in buffer A (50 mM MES-NaOH, pH=6.5, 20% glycerol, 5 mM CaCl 2 , 5 mM MgCl 2 and 1 mM of a mixture of protease inhibitors containing amino caproic acid, benzamidine and phenylmethyl sulphonyl fluoride), and were broken, at 4 °C, by the application of five Bead Beater (Biospec Products) cycles (20 s blend and 5 min pause), using 0.1–1.0 mm glass beads. Following the separation of the broken cells from the beads, intact cells and cell debris were removed from the green solution by centrifugation for 2 min at 2,000 r.p.m. The thylakoid membranes were precipitated from the obtained supernatant by an ultra centrifugation at 35,000 r.p.m. in a Ti-50 rotor for 20 min. The green pellet was washed twice in buffer B (buffer A containing an additional 5 mM CaCl 2 ) and separated by centrifugation at 35,000 r.p.m. PSII was extracted and purified by homogenizing the thylakoids in buffer C (40 mM MES-NaOH, pH=6.0, 5% glycerol and 0.02% n -dodecyl β- D -maltoside) to a chlorophyll concentration of 1.6 mg ml −1 . n -Dodecyl β- D -maltoside was added to a final concentration of 0.6% and the solution was stirred at room temperature for 20 min. Following 100 min of ultra centrifugation at 50,000 r.p.m. in a Ti-70 rotor (at 4 °C), the resulting supernatant was filtrated through a 0.45-μm filter, and to the filtrated solution, an equivalent volume of 24% of buffer D (buffer C containing 50 mM MgSO 4 ) was added. The solution was loaded (15 ml min −1 ) onto a TSK Toyo Pearl DEAE 650 anion exchange fast protein liquid chromatography column (2.5×35 cm 2 ), prewashed with 24% buffer D ( Supplementary Fig. S1) . The loaded column was washed in the AKTA explorer (Amersham Pharmacia Biotech) with 2 column volumes (CVs) 24% of buffer D. Following an isocratic step to 50% buffer D (0.5 CV), a linear gradient from 50 to 80% buffer D was run in 3 CVs. The column was then washed with 3.5 CVs of 100% B. The elution from the column was performed at 10 ml min −1 . The phycobiliproteins (PBPs) were eluted from the column during the wash step and the PSII was obtained at a sharp elution peak at 50–65% buffer D. PSI was eluted from the column at the highest MgSO 4 concentration applied (100% buffer B). The obtained PSII and PSI were analysed by: ultraviolet–visible spectroscopy ( Supplementary Fig. S2) ; Deriphat NativePAGE ( Supplementary Fig. S3) ; and SDS–PAGE, in which the different complexes were fully denatured ( Supplementary Fig. S4) . Supplementary Fig. S2 indicates that the PSII spectrum (red trace) demonstrates a 673-nm absorption peak, whereas the PSI spectrum (blue trace) exhibits a 680-nm peak. The latter indicated that the separated PSII and PSI complexes were highly pure. To further characterize it, native and denatured PAGE analyses were performed. The native 6% acrylamide gel was electrophorized in the presence of Deriphat. Supplementary Fig. S3 indicates that when the gel is subjected to ultraviolet light, the PSII (both in its monomeric (m) and dimeric (d) forms) is highly fluorescent, whereas the obtained trimeric (t) PSI has no fluorescence. Although the native gel further demonstrated the high purity of each of the complexes, the most solid proof was obtained with denatured PAGE using 12.5% acrylamide. Supplementary Figure S4 clearly indicates that the PSII complex contains the typical subunits of PSII (for example, CP47, CP43, D1, D2 and so on), whereas PSI contains its typical subunits (for example, PsaA/B, PsaD and so on). Moreover, as Supplementary Fig. S4 indicates, no cross contaminations between the two complexes exist. The pure PSII complexes were used to construct the photo-bioelectrochemical cells. Modification of the electrodes pMBQ/PSII-modified Au electrodes: clean Au-coated glass slides (from Nunc International, Rochester, USA) were reacted with an aqueous solution of MBQ, 10 mM, for 5 h. Electropolymerization of MBQ, 0.2 mg ml −1 dissolved in phosphate buffer, PB (0.1 M, pH=7.4), was then performed on the MBQ-functionalized slides by the application of a constant potential, E =0.6 V versus SCE, for fixed time-intervals. Following the electropolymerization process, the electrodes were washed with PB and reacted with 100 μl of PSII (1 mg chl ml −1 ). The resulting pMBQ/PSII-modified electrodes were crosslinked with BS 3 , 0.01 mg ml −1 , for 30 min and washed with PB. Bis-aniline-crosslinked Au NPs/PSII electrodes: clean Au-coated glass slides were reacted with p -aminothiophenol, 10 mM, in ethanol for 5 h. The thioaniline-functionalized slides were, then, subjected to electropolymerization in the presence of the thioaniline-modified Au NPs, using a fixed number of repetitive cyclic voltammetry scans, ranging between −0.1 and 1.1 V versus SCE, and at a scan rate of 100 mV s −1 . Following the electropolymerization process, the electrodes were washed with PB and reacted with PSII (1 mg chl ml −1 ). The resulting electrodes were crosslinked with BS 3 for 30 min and washed with PB. BOD/CNTs-modified GC electrodes: SWCNTs, 10 mg ml −1 , were dispersed in dimethylformamide to yield a stable suspension. The dispersion, 5 μl, was deposited onto polished GC electrodes to generate the CNTs-modified GC electrode. A BOD solution (5 μl, 0.14 mg ml −1 ) in HEPES buffer (0.1 M, pH=7.2) was deposited on the electrodes, and after 30 min, 1 μl of BS 3 , 0.01 mg ml −1 , was added. The electrodes were then allowed to dry in air. Electrochemical characterization of the electrodes The redox potential of the pMBQ-modified electrode was determined by cyclic voltammetry. The linear relationship between the anodic peak current and the scan rate, confirmed the confinement of the polymer to the electrode (see Supplementary Fig. S5 ). The bioelectrocatalytic functions of the BOD/CNTs-modified GC cathode were characterized by following the electrocatalytic cathodic currents in the presence of O 2 , using cyclic voltammetry (for the experimental results, see Supplementary Fig. S6 ). Measurements and instrumentation Electrochemical measurements were performed using an Autolab potentiostat (ECO Chemie, The Netherlands) driven by GPES software. A KCl-saturated SCE (or a Ag wire) and a carbon rod ( d= 5 mm) were used as the reference and counter electrodes, respectively. Photoelectrochemical measurements were performed using a home-built system that included a Xe lamp (Oriel, model 6258, P =300 W), a monochromator (Oriel, model 74000, 2 nm resolution) and a chopper (Oriel, model 76994). The electrical output from the cell was sampled by a lock-in amplifier (Stanford Research, model SR 830 DSP). The shutter-chopping frequency was controlled by a Stanford Research pulse/delay generator, model DG535. The photogenerated currents were measured between the modified Au working electrode and a Pt plate counter electrode. The quantum efficiency was evaluated by measuring the generated photocurrents and the light power absorbed by the respective PSII-modified electrodes. The absorbed light power, P , was determined by subtracting the sum of powers associated with the light transmitted through the gold-coated glass slides modified with the polymerized layers and the PSII units, and the light power reflected from these surfaces, from the incident lamp power. The absorbed light power was also corrected for gold surfaces modified with the polymeric assemblies but in the absence of the PSII units. Substitution of the measured photocurrent, I, and the absorbed light power, P , in equation (1) yields the photocurrent quantum yield. Where h is Planck's constant, c is the vacuum velocity of light, λ is the selected wavelength of light and e is the charge of an electron. In one experiment, the Autolab potentiostat was coupled to the photoelectrochemical apparatus, allowing the measurement of the photocurrents upon the application of different external potentials on the bis-aniline-crosslinked Au NPs/PSII electrode (see Supplementary Fig. S7 ). For the PBFC measurements, the BOD/CNTs-modified GC cathode and the respective anode (pMBQ/PSII or bis-aniline-crosslinked Au NPs/PS-II) were placed into a 10 ml cell that was filled with PB (0.1 M, pH=7.4). The biofuel discharge (polarization) curves were recorded under air (or nitrogen) at variable external resistances, and by using an electrometer (Keithley 617). In these experiments, the light source was an optical fibre (Fiber Lite, model 190, P ~0.1 W) by Dolan-Jenner. Quartz-crystal microbalance measurements were performed using a home-built instrument linked to a frequency analyser (Fluke) and using Au quartz crystals (AT-cut, 10 MHz). How to cite this article: Yehezkeli, O. et al . Integrated photosystem II-based photo-bioelectrochemical cells. Nat. Commun. 3:742 doi: 10.1038/ncomms1741 (2012).